Unbounded number of channel uses may be required to detect quantum capacity Transmitting data reliably over noisy communication channels is one of the most important applications of information theory, and is well understood for channels modelled by classical physics. However, when quantum effects are involved, we do not know how to compute channel capacities. This is because the formula for the quantum capacity involves maximizing the coherent information over an unbounded number of channel uses. In fact, entanglement across channel uses can even increase the coherent information from zero to non-zero. Here we study the number of channel uses necessary to detect positive coherent information. In all previous known examples, two channel uses already sufficed. It might be that only a finite number of channel uses is always sufficient. We show that this is not the case: for any number of uses, there are channels for which the coherent information is zero, but which nonetheless have capacity. In the classical case, not only can we exactly characterize the maximum rate of communication over any channel—its capacity—we also have practical error-correcting codes that attain this theoretical limit. It is instructive to review why the capacity of classical channels is a solved problem. Even though optimal communication over a discrete, memoryless classical channel involves encoding the information across many uses of the channel, Shannon showed that a channel’s capacity is given by optimizing an entropic quantity (the mutual information) over a single use of the channel. This follows immediately from the fact that mutual information is additive. It is for this reason that additivity questions for quantum channel capacities took on such importance, and why the major recent breakthroughs proving that additivity is violated [1] , [2] had such an impact. A regularized expression for the quantum capacity has been known for some time [3] , [4] , [5] —the optimization of an entropic quantity (the coherent information I coh ) in the limit of arbitrarily many uses of the channel: Here where is a channel from A to B, ρ AR is a purification of ρ A , and S denotes the von Neumann entropy. However, the regularization renders computing the quantum capacity infeasible; it involves an optimization over an infinite parameter space. Were the coherent information additive, so that , the regularization could be removed and the quantum capacity could be computed by a single optimization, similarly to classical channels. However, this is not the case. The first explicit examples of superadditivity were given by Di Vincenzo et al. [6] , and extended by Smith et al. [7] . For these examples (where is a particular depolarizing channel) it was shown (numerically) that for small values of n ≤33. While the classical capacity of quantum channels also involves a regularized formula [2] , we at least know precisely in which cases it is zero: simply for those channels whose output is completely independent of the input. The set of channels with zero quantum capacity is much richer. Indeed, the complete characterization of such channels is unknown. To date, we know of only two kinds of channels with zero quantum capacity: antidegradable channels [8] , [9] and entanglement-binding channels [10] . The former has the property that the environment can reproduce the output, thus Q =0 by the no-cloning theorem [11] . The latter can only distribute PPT entanglement, which cannot be distilled by local operations and classical communication [12] , again implying Q =0. This has marked consequences. It is possible to take two channels with no quantum capacity whatsoever ( ), antidegradable and entanglement-binding, which, when used together, do have quantum capacity ( ). This ‘superactivation’ phenomenon was discovered recently by Smith and Yard [1] (and extended in ref. 13 ). They also show that a single-channel , which can be ‘switched’ between acting like or , exhibits an extreme form of superadditivity of the coherent information, where . Even stronger superactivation phenomena have been shown in the context of zero-error communication [14] , [15] , [16] , [17] , [18] . These recent additivity violation results demonstrate how much we still do not understand about the behaviour of information in quantum mechanical systems. On the one hand, it means that the known formula for the quantum capacity must be regularized, hence cannot be used to compute the capacity. On the other hand, since the coherent information is additive for unentangled input states, additivity violation also implies that entanglement can protect information from noise in a way that is not possible classically. But just how badly can additivity be violated? One might hope that, at least in determining whether the quantum capacity is non-zero, one need only consider a finite number of uses of a channel. Indeed, since the Smith and Yard construction relies on combining the only two known types of zero-capacity channels, one might dare to hope that even two uses suffice. (Similarly, for the classical capacity of quantum channels the only known method for constructing examples of additivity violation [2] , [19] cannot give a violation for more than two uses of a channel, and there is some evidence that this may be more than just a limitation of the proof techniques [20] .) Were this the case, one could decide if a channel has quantum capacity by optimizing the coherent information over two uses of the channel, which is not substantially more difficult than the optimization over a single-channel use. In this paper, we show that this is not the case: additivity violation is essentially as bad as it could possible be. More precisely (see Fig. 1 ), we prove that for any n one can construct a channel for which the coherent information of n uses is zero ( ), yet for a larger number of uses the coherent information is strictly positive, implying that the channel has non-zero quantum capacity ( ). We also prove that there can be a gap between and the quantum capacity for an arbitrarily large number n of uses of the channel. Our result implies that, in general, one must consider an arbitrarily large number of uses of the channel just to determine whether the channel has any quantum capacity at all. 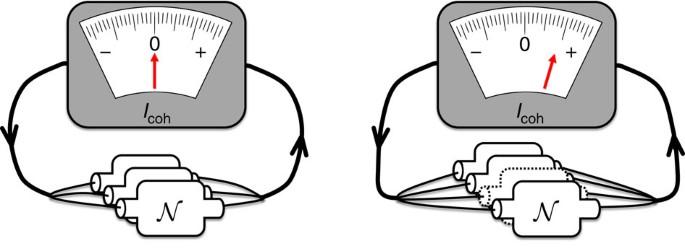Figure 1: Positive coherent information can be detected after unbounded uses. Checking the coherent information (Icoh) forn=3 uses fails to reveal that channelhas quantum capacity. However, the channel has capacity and this can be shown by checking some larger number of uses of the channel. We show that for any number of uses of the channelnthere are channels with this behaviour. Figure 1: Positive coherent information can be detected after unbounded uses. Checking the coherent information ( I coh ) for n =3 uses fails to reveal that channel has quantum capacity. However, the channel has capacity and this can be shown by checking some larger number of uses of the channel. We show that for any number of uses of the channel n there are channels with this behaviour. Full size image A channel with zero coherent information but positive capacity Perhaps the earliest indication that deciding whether a channel has quantum capacity may be difficult comes from the work of Watrous [21] , who showed that an arbitrarily large number of copies of a bipartite quantum state can be required for entanglement distillation assisted by two-way classical communication. Our result can be regarded as the counterpart of [21] for the quantum capacity (which is mathematically equivalent to entanglement distillation assisted by one-way communication). However, since the proof ideas and techniques of [21] assume two-way communication, they do not apply in our setting. Our result is instead based on the ideas of Smith and Yard, in particular the intuition provided by Oppenheim’s commentary thereon [22] . This intuition comes from a class of bipartite quantum states called pbits (private bits) [23] , together with the standard equivalences between quantum capacity (sending entanglement over a channel) and distilling entanglement from the state obtained by sending one half of a maximally entangled state through the channel (its Choi–Jamiołkowski state). A pbit ρ aAbB is a state shared between Alice (who holds aA) and Bob (who holds bB), where the ab part of the system is usually called the ‘key’, AB the ‘shield’ (see Fig. 2 for a graphical representation and refer to ‘Channel Construction’ in the Supplementary Note 1 for the mathematical details of the pbit construction). 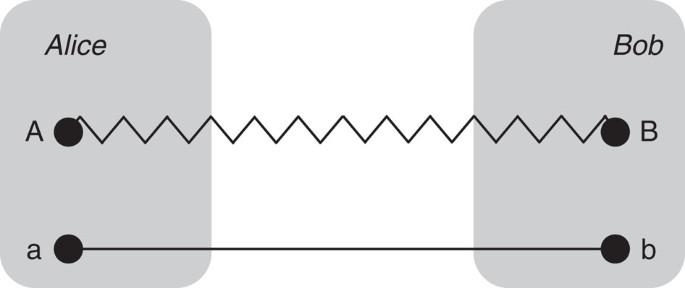Figure 2: Pbit representation. A pbit is a bipartite state with subsystems ab called the “key” and AB called the “shield”. One party, Alice, holds the subsystems aA and the other party, Bob, holds the subsystems bB For concreteness let us consider a state ρ aAbB of the following form: Figure 2: Pbit representation. A pbit is a bipartite state with subsystems ab called the “key” and AB called the “shield”. One party, Alice, holds the subsystems aA and the other party, Bob, holds the subsystems bB Full size image That is, they hold one of the two states with equal probability. Here are Bell states and σ ± are hiding states [24] encoding the identity of the Bell state. Hiding states are perfectly distinguishable globally, but cannot be distinguished locally using local operations and classical communication. If Alice and Bob knew which Bell state they held, they would have at least one ebit of shared entanglement. But this information, and hence the entanglement, is inaccessible to them unless one party is given the whole-shield AB. Now imagine they have access to a quantum erasure channel which with probability 1/2 transmits its input perfectly, but otherwise completely erases it. It is well known that such a channel cannot be used to transmit any entanglement [25] . However, if they also share ρ aAbB , Alice can use the erasure channel to send her part A of the shield to Bob. If the erasure channel transmits, Bob now holds the entire AB system and can now distinguish σ ± . Thus, with probability 1/2, Alice and Bob can now extract the entanglement from ρ aAbB . Instead of supplying Alice and Bob with the state ρ aAbB and an erasure channel, we supply them with a switched channel. This has an auxiliary classical input that controls whether the channel acts as or Γ, where Γ is the channel with Choi–Jamiołkowski state ρ aAbB . The above argument then implies that no quantum information can be sent over a single use of the channel, but it can be sent using two uses, by switching one to and the other to Γ. This is the intuition behind the Smith and Yard construction [22] . However, it is constructed out of two very particular types of quantum channels, so this idea does not seem to extend to more than two channel uses. Nonetheless, the intuition behind our result is based on a refinement of these ideas, which we now sketch. Sketch of the general construction We want to achieve two seemingly contradictory goals: Firstly, to prevent Alice from sending any quantum information to Bob over n of uses of the channel, and secondly to permit this when Alice has access to some larger number of uses N > n . We can achieve the first goal by increasing the erasure probability of the erasure channel to something much closer to one, and also adding noise to the Γ channel; the noise then swamps any entanglement. The problem is that this seems to render the second goal impossible. If the channel is so noisy that it destroys all entanglement sent through it, then no amount of coding over multiple uses of the channel can transmit any quantum information. However, note that the information that Alice needs to send to Bob in order to extract entanglement from the pbit ρ aAbB is essentially classical. Bob just needs to know one classical bit of information to distinguish the two hiding states. This suggests that classical error correction might help Alice send this information to Bob, even when the channel is very noisy. The intuition behind our proof is that a simple classical repetition code suffices. Instead of the pbit ρ aAbB , we use a pbit that contains N copies of the shield. For Bob to distinguish the hiding states, it suffices for a single copy to make it through the erasure channel. Alice now tries to send all of the copies of the shield through many uses of the erasure channel. However high the erasure probability, the probability that at least one will get through becomes arbitrarily close to one for sufficiently many attempts. Making the above intuition rigorous is non-trivial: first, we must prove that the coherent information of n uses of the channel is strictly zero, for any input to the channel (not just the input states from the above intuition). To this end, we cannot directly use a pbit with N -copy shield of the form given above, as it would have distillable entanglement. We must instead adapt an approximate pbit construction from [23] . However, we must then take this approximation into account in the proof that the channel does have capacity. This requires a delicate analysis of the various parameters of our channel to show that both of the desired properties can hold simultaneously, which requires a more technical argument described in the Methods section (with full technical details in the Supplementary Note 1 ). A natural question, which we leave open, is whether a stronger form of the result holds, which gives a constant upper bound on the channel dimension. It is even conceivable that the presence of quantum capacity is undecidable, which would imply the stronger form of result mentioned. It would also be interesting to see if one can obtain a result analogous to ours for the private capacity of quantum channels. Channel description First, let us give a more precise description of our channel. The erasure channel with erasure probability p is where, is the identity channel from A to B, and F is the erasure flag. The channel Γ aA→bB will belong to the class of PPT entanglement-binding channels whose Choi–Jamiołkowski state is an approximate pbit [23] . We show that Γ can be constructed with and consisting of N parts, such that even if Bob only receives part A i of Alice's shield for any i , they obtain close to one ebit of one-way distillable entanglement. With the shorthand , and , let be a noisy version of the channel Γ. More precisely, a composition of Γ with an erasure channel: Our construction uses channels of the form Here projects onto the i th computational basis vector of the qubit system S, which thereby acts as a classical switch allowing Alice to choose whether the channel acts as p or on the main input . S is retained in the output, which lets Bob learn which choice was made. Proof outline We now state and outline the proof of our main result—for any number of channel uses there exists a channel with positive capacity but zero coherent information. Formally, we prove the following: Theorem. Let be the channel defined in equation (8). For any positive integer n , if κ ε(0, 1/2) and p ε[(1+ κ n ) −1/ n ] then we can choose N and Γ such that: The proof is divided in two parts. We first prove that, given n and κ , for any Γ with zero capacity there is a range of p that makes the coherent information of zero. In the second part we prove that there exists Γ with zero capacity such that has positive capacity. For the first part we can simplify the analysis of by showing that it is optimal to make a definite choice (that is, a computational basis state input) for each of the n switch registers. For each possible setting of the n switches, the coherent information is a convex combination of the coherent information for three cases, weighted by their probabilities: every channel erases, all of the p erase but not all erase and at least one of the p does not erase (and therefore acts as the identity channel). The coherent information for second and third cases can be upper bounded, respectively, by zero and H (R), where R is a system that purifies the input. For the first case it is bounded above by − H (R). Weighting by the probabilities, we find that the total coherent information is upper bounded by (1−(1+ κ n ) p n ) H (R). For any n and κ we can therefore find p such that this upper bound is zero. To prove the second part, we show that for fixed κ , p we can find a Γ with an N -copy shield such that the coherent information of N +1 uses of the channel is positive for some N +1> n . We number the channel uses 0, …, N and label the systems involved in the i th use of the channel with superscript i . Consider the following input. The switch registers are set to select for use 0 and p for the remaining uses 1, …, N . We maximally entangle subsystem of (which is acted on by ) with subsystem of (acted on by an erasure channel). We also maximally entangle subsystem a 0 of with a purifying reference system, which is retained by Alice. The remaining input subsystems are set to an arbitrary pure state. The resulting coherent information is a convex combination of cases where erases, does not erase but all the p erase, and and at least one p do not erase. The first case contributes coherent information −1 weighted by its probability κ. The second case contributes approximately zero coherent information (due to a standard property of pbits). In the third case, after channel use 0, Alice and Bob share the Choi–Jamiołkowski state of Γ on systems , and after the N uses of p at least one of reaches Bob unerased. They then share a state with close to one ebit of one-way distillable entanglement (coherent information +1). This contribution is weighted by the probability (1− κ )(1− p N ). We show that for p ε(0, 1), κ ε(0, 1/2), we can find a Γ with large enough N for which the overall coherent information is positive, proving that . Further mathematical details are given in the Supplementary Note 1 . How to cite this article: Cubitt, T. et al. Unbounded number of channel uses may be required to detect quantum capacity. Nat. Commun. 6:6739 doi: 10.1038/ncomms7739 (2015).